Determination of monolayer-protected gold nanoparticle ligand–shell morphology using NMR It is accepted that the ligand shell morphology of nanoparticles coated with a monolayer of molecules can be partly responsible for important properties such as cell membrane penetration and wetting. When binary mixtures of molecules coat a nanoparticle, they can arrange randomly or separate into domains, for example, forming Janus, patchy or striped particles. To date, there is no straightforward method for the determination of such structures. Here we show that a combination of one-dimensional and two-dimensional NMR can be used to determine the ligand shell structure of a series of particles covered with aliphatic and aromatic ligands of varying composition. This approach is a powerful way to determine the ligand shell structure of patchy particles; it has the limitation of needing a whole series of compositions and ligands' combinations with NMR peaks well separated and whose shifts due to the surrounding environment can be large enough. Gold nanoparticles, composed of a metallic core and a self-assembled monolayer (SAM) of thiolated molecules (the ligand shell), have multiple potential applications, for example, sensing, catalysis, drug delivery and molecular recognition [1] , [2] , [3] , [4] , [5] , [6] . The chemical functionality of ligand molecules determines most of the nanoparticles' interface-related properties [7] . Mixtures of ligand molecules are often used to coat the nanoparticles [8] , [9] . Typically, this is done so that each of the ligand shell components provides a different property to the nanoparticles. Recently, it has become apparent that the organization of the molecules in the ligand shell can also affect the particles' overall behaviour. Particles coated with a mixture of the molecules in a random arrangement (random mixture) will tend to show properties that are averages of the properties of each ligand molecule. Janus particles preserve the ligand properties but show unique collective behaviours, for example, assembling in unique structures [10] . There are many predictions for unique properties of patchy particles that are particles with multiple small domains in their ligand shell [11] . Our group has found that binary mixtures of dislike ligands differing in length self-assemble into stripe-like domains of alternating composition on the particles' ligand shell [12] , [13] , [14] . This morphology is key in determining the particles interaction with cell membranes [15] , [16] , [17] , provides unique solubility and interfacial properties [18] , [19] and helps with the particles' properties in catalysis and molecular recognition [20] , [21] . Despite the importance of the ligand shell structure, current methods for determining the pattern of ligand phase separation on nanoparticles are challenging and time consuming. It is possible to determine whether the ligand shell of nanoparticle is randomly mixed or phase separated using infrared spectroscopy [22] , electron spin resonance [23] , mass spectroscopy [24] , transmission electron microscopy (TEM) [25] or fluorescence [26] . All of these methods require accurate data interpretation, and work only for a subset of particles. None can determine the pattern of surface morphology of the ligand shell in the case of phase separation. When the occurrence of Janus particles is suspected, it is possible to use mass spectroscopy [24] , contact angle measurements [27] or two-dimensional (2D) NMR to test the hypothesis [28] . The occurrence and structure of patchy particles are hard to characterize. To the best of our knowledge, the only method capable to determine the morphology of the ligand shell of particles is scanning tunnelling microscopy (STM). Unfortunately, it is based on extensive comparative analysis of multiple images obtained at different tip speeds and on different samples [12] . Sample preparation itself, with its requirement of cleanness, nanoparticles purity, and good distribution and coverage over the entire sample surface, is a major challenge [29] , [15] . Importantly, although STM can identify a sample that has stripe-like [29] or Janus [30] (see also: Reguera, Pons, Glotzer, Stellacci unpublished results) domains, in the cases where STM images fail to show any structure, little can be stated on the ligand shell structure. Here, we present a comprehensive but simple method to determine nanoparticles' ligand shell structure based on the most common characterization technique for organic chemists: NMR. Our method is based on analysing 1D and 2D 1 H NMR spectra of particles coated with a binary mixture of aliphatic and aromatic ligand molecules of varying composition and can be applied in all those cases where some of the peaks of the molecules used are well separated, with environment caused shifts large enough. Key assumptions As illustrated in Fig. 2, when plotting the peak position for a generic proton NMR as a function of composition, different trends are theoretically possible depending on the ligand shell structures [31] . In the case of random mixtures, the average composition of the first nearest neighbors' shell (FNN) for any molecule coincides with the overall composition of the ligand shell. As a consequence, a linear trend with composition will be observed (Fig. 2a), because the chemical shift for the proton is sensitive to the surroundings. If we call B the shift of a generic NMR peak for molecules in 'bulk' phase that is surrounded by similar molecules, and I the shift for molecules at an interface with different molecules, it is trivial to show that in this case the shift F of a nanoparticles of composition x A is: This coincidence between local and global compositions is removed in the case of phase separation. For Janus particles only the ligands at the two-component interface have a mixed composition in FNN whereas all of the others have the same FNN composition of homoligand nanoparticles. Assuming that the 'interfacial' region in such particles is a stripe of constant thickness t then one can rigorously derive (see Methods) the following dependence of F on x A : with r being the particles core radius. Equation (2) shows a 1/ x A trend for the chemical shift (Fig. 2b). For patchy particles, the relationship is more complex (given that the shape of the patches does change with composition) and it leads to a sigmoidal trend whose analytical shape will strictly depend on the shape evolution of the domains. Similar considerations should hold for any form of spectroscopy with modes sensitive to the surroundings. Our group tested part of this theory [31] with Fourier transform infrared spectroscopy finding a linear dependence of the CH stretching modes on composition for randomly mixed ligand shells and a sigmoidal one for striped particles [22] . NMR offers valuable insights beyond what linear spectroscopy can provide. 2D NMR, nuclear Överhauser enhancement spectroscopy (NOESY) allows for the determination of average proximity between nuclei. NOESY is a 2D NMR technique that exhibits cross-peaks arising from dipole–dipole interaction (that is, through-space coupling) between nuclear spins that are close enough in proximity (typically <0.4 nm). The intensity of a NOESY cross-peak depends inversely on the sixth power of the distance of protons, so this technique can be exploited for an estimation of internuclear distance. For nanoparticle samples, the presence of cross-peaks can be used as a proof that the distance between two ligands is <0.4 nm. In Fig. 2, we illustrate what happens to cross-peaks between protons of the two different ligand molecules in the case of the various morphologies possible on nanoparticles. For random mixtures, strong cross-peaks are expected as each kind molecule is in the FNN shell of the other type of molecules. In the case of Janus particles, this occurs only for the few interfacial molecules hence basically cross-peaks are not expected. For patchy particles, (specifically in the case of patches with at least one characteristic dimension being small) strong cross-peaks are expected. Here, we postulate and show that a combination of 1D and 2D NMR is a fingerprint to distinguish randomly mixed, Janus and patchy particles. NMR on nanoparticles NMR has been routinely used to determine the structure of organic materials, including ligand molecules on nanoparticles, because NMR shifts change on the perturbation of the magnetic field at the nucleus that is sensitive to the surrounding electrons. Previous research of NMR on nanoparticle samples discussed the nature of line broadening [32] , [33] , [34] , the effect of particle size on NMR frequency ( F ) [35] , [36] and the dependency of line width and F to the nuclei distance from nanoparticle surface [37] . As SAMs of thiol ligands at the surface of gold nanoparticles are tightly packed, their NMR F is not only determined by the chemical structure of themselves but also affected by neighbouring ligands. The subtle change in chemical shift reflects the surrounding environment of ligands. Malicki et al . [38] have observed an upfield shift (towards smaller chemical shift) of aromatic ligands in 1 H NMR when they self-assemble on nanoparticles, and that the shift is dependent on the packing density and the neighbouring environment of ligands. The upfield shift of aryl protons is caused by the ring currents from proximal arene rings. Therefore, we chose a solely aromatic ligand diphenyl thiol (DPT), 1 , together with aliphatic ligand dodecanethiol (DDT), 2 , or 3,7-dimethyloctanethiol (DMOT), 3 , as a model to study the morphology of mixed SAMs on gold nanoparticles. In addition, the fact that their 1 H NMR peaks are well separated provides the ease and cleanness for data analysis. The structures of DPT, DDT and DMOT molecules are shown in Fig. 1 . Gold nanoparticles were synthesized through the Stucky method using thiol mixtures of varying stoichiometric ratios [39] . We stress that the actual ligand composition on nanoparticles was determined by 1 H NMR after decomposing the gold core via cyanide etching [40] using the ratio between the integration the aromatic peaks from DPT and that of methyl from DDT (see Supplementary Fig. S1 for a representative NMR spectrum obtained after cyanide decomposition). Particle size was analysed by TEM. To acquire accurate NMR signal of the ligand shell of nanoparticles, it is of great importance to thoroughly remove all free ligands that are physically adsorbed. Many methods including repeated ultrasonication/centrifugation, dialysis and filtration were used to completely clean the nanoparticles. After cleaning, nanoparticles were dissolved in CD 2 Cl 2 at 5.0 mg ml −1 and analysed by NMR. All spectra were processed by Topspin 2.1 and calibrated by the CD 2 Cl 2 solvent peak. No peaks of free ligands could be seen, indicating the cleanness of nanoparticles. In a few spectra there exists a relatively sharp and small peak at 7.36 p.p.m. We believe this is not because of free ligands—this feature is discussed below. The centre of the broad peak was calculated by Gaussian–Lorentzian fitting of the spectra and statistically analysed by multiple measurements on multiple samples made on many different days. It is important to notice that in Fig. 3d–f, each data point is the average value of NMR chemical shifts calculated from at least three samples, and the error bars represent the largest standard deviation (s.d. ), the compositional error bars are the s.d. 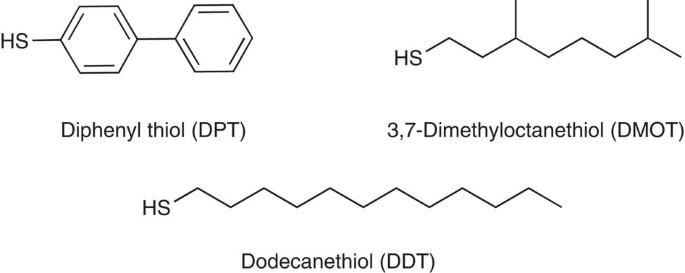Figure 1: The ligand molecules adopted for this study. DPT, DMOT and DDT. of DPT percentage in the ligand shell, calculated on three different samples (see Table 1 for complete data entries used for the calculation). Figure 1: The ligand molecules adopted for this study. DPT, DMOT and DDT. Full size image Table 1 Calculation of number of ligands at the poles. Full size table Randomly mixed nanoparticles Mixtures of DPT and DMOT are expected to form random mixtures when coating nanoparticles given that DMOT, due to its branched structure, should not have an ordered crystalline arrangement on nanoparticles and hence little enthalpy of phase separation relative to another ligand [14] . This finding is partly supported by the lack of any detectable structure in STM images of these particles (Fig. 3j) [14] , [16] . NMR result strongly confirms this type of structure. In fact, Fig. 3a shows the superimposed spectra of representative nanoparticles Au-DPT 0.22 DMOT 0.78 , Au-DPT 0.60 DMOT 0.40 and Au-DPT 0.82 DMOT 0.18 in the aromatic region (see Supplementary Fig. S5 for full spectra of all compositions). The broad peak gradually shifts upfield (towards small chemical shift) when the fraction of DMOT increases from 22 to 60% and to 82% (Fig. 3a). As these particles are very similar in size and only differ in ligand composition, the NMR peak shift must be a result of how the two ligands arrange on nanoparticles. The shift of peak centre is linear as a function of ligand composition (Fig. 3d, linear fit, y =7.47–0.00448 x , R 2 =0.974), as expected from equation (1). In addition to the investigation on nanoparticles' 1D 1 H NMR, experiments of NOESY were carried out. Figure 3g shows the NOESY spectra of representative Au-DPT 0.40 DMOT 0.60 particles (see Supplementary Fig. 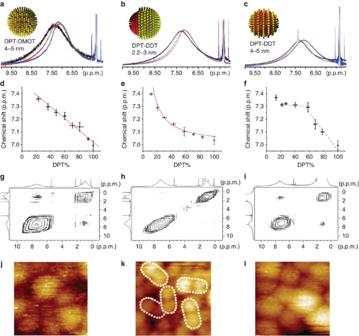Figure 3: NMR and STM images of nanoparticles. (a)1H NMR of randomly mixed nanoparticles Au-DPT0.22DMOT0.78(black), Au-DPT0.60DMOT0.40(red) and Au-DPT0.82DMOT0.18(blue). (b)1H NMR of Janus nanoparticles Au-DPT0.19DDT0.81(black), Au-DPT0.56DDT0.44(red) and Au-DPT0.82DDT0.18(blue). (c)1H NMR of striped nanoparticles Au-DPT0.21DDT0.79(black), Au-DPT0.58DDT0.42(red) and Au-DPT0.78DDT0.22(blue). (d–f) Chemical shift of1H NMR as a function of alkanethiol percentage for randomly mixed, Janus and striped nanoparticles, respectively. Solid red lines in (d) and (e) are the fit to the data (see text). Error bars represent the s.d. of the mean of the chemical shift and of the DPT percentage calculated after cyanide decomposition. (g–i–) NOESY spectra of randomly mixed nanoparticle Au-DPT0.40DMOT0.60, Janus nanoparticle Au-DPT0.56DDT0.44and striped nanoparticle Au-DPT0.58DDT0.42, respectively. (j–l) STM image of randomly mixed nanoparticle Au-DPT0.40DMOT0.60, Janus nanoparticle Au-DPT0.56DDT0.44and striped nanoparticle Au-DPT0.58DDT0.42, respectively. (j) and (l) are (17×17 nm) while (k) is (20x20 nm). White dotted ovals delimit each single Janus nanoparticle. Larger STM images can be found inSupplementary Material,Supplementary Figs S2 and 3. S6 for spectra of all compositions). These particles show clearly NOESY cross-peaks suggesting a close proximity of the two ligands. Overall, the agreement between the predicted ( Fig. 2 ) and measured ( Fig. 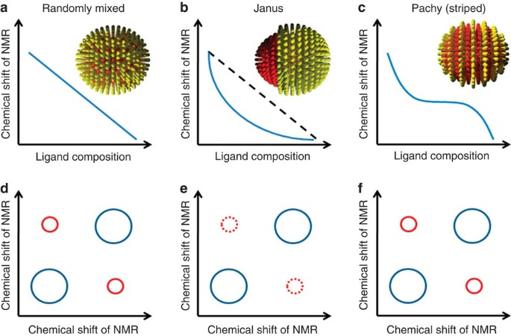3 ) 1D and 2D NMR spectra for random packing is remarkable. Figure 2: Idealized NMR plots for nanoparticles coated with binary mixtures of ligands. (a–c) Chemical shift of NMR as a function of ligand composition for randomly mixed, Janus and patchy (striped) nanoparticles, respectively. (d–f) NOESY of randomly mixed, Janus and patchy (striped) nanoparticles, respectively. Figure 2: Idealized NMR plots for nanoparticles coated with binary mixtures of ligands. ( a – c ) Chemical shift of NMR as a function of ligand composition for randomly mixed, Janus and patchy (striped) nanoparticles, respectively. ( d – f ) NOESY of randomly mixed, Janus and patchy (striped) nanoparticles, respectively. Full size image Figure 3: NMR and STM images of nanoparticles. ( a ) 1 H NMR of randomly mixed nanoparticles Au-DPT 0.22 DMOT 0.78 (black), Au-DPT 0.60 DMOT 0.40 (red) and Au-DPT 0.82 DMOT 0.18 (blue). ( b ) 1 H NMR of Janus nanoparticles Au-DPT 0.19 DDT 0.81 (black), Au-DPT 0.56 DDT 0.44 (red) and Au-DPT 0.82 DDT 0.18 (blue). ( c ) 1 H NMR of striped nanoparticles Au-DPT 0.21 DDT 0.79 (black), Au-DPT 0.58 DDT 0.42 (red) and Au-DPT 0.78 DDT 0.22 (blue). ( d – f ) Chemical shift of 1 H NMR as a function of alkanethiol percentage for randomly mixed, Janus and striped nanoparticles, respectively. Solid red lines in ( d ) and ( e ) are the fit to the data (see text). Error bars represent the s.d. of the mean of the chemical shift and of the DPT percentage calculated after cyanide decomposition. ( g–i –) NOESY spectra of randomly mixed nanoparticle Au-DPT 0.40 DMOT 0.60 , Janus nanoparticle Au-DPT 0.56 DDT 0.44 and striped nanoparticle Au-DPT 0.58 DDT 0.42 , respectively. ( j–l ) STM image of randomly mixed nanoparticle Au-DPT 0 . 40 DMOT 0.60 , Janus nanoparticle Au-DPT 0.56 DDT 0.44 and striped nanoparticle Au-DPT 0.58 DDT 0.42 , respectively. ( j ) and ( l ) are (17×17 nm) while ( k ) is (20x20 nm). White dotted ovals delimit each single Janus nanoparticle. Larger STM images can be found in Supplementary Material , Supplementary Figs S2 and 3 . Full size image Janus nanoparticles Theory [14] and experiments [30] predict that very small particles coated with binary mixtures of dislike ligand molecules have a ligand morphology that is dictated by the enthalpy of phase separation. Hence, for two molecules known to form ordered arrangement on nanoparticles as DPT and DDT, one would expect that two macro domains would form, this arrangement (Janus) would minimize domain boundaries hence minimizing the enthalpy (and consequently free energy) of the system. We have previously determined and recently confirmed that for molecules such as terphenylthiol (TPT) and DDT this enthalpy-dominated system occur for particles with a core diameter <2 nm (ref. 30 ). For this reason, we synthesized DPT/DDT-coated particles of ~2 nm in diameter. On such small nanoparticles (see Supplementary Fig. S7 form TEM) Janus morphology is consistent with what observed by STM ( Fig. 3k ). The result of NMR investigation of these Janus particles is shown in Fig. 3b,e and Supplementary Fig. S8 . In Fig. 3b , NMR spectra of Au-DPT 0.56 DDT 0.44 and Au-DPT 0.82 DDT 0.18 are similar, whereas the peak of Au-DPT 0.19 DDT 0.81 appears in a downfield region. The dependence of the peak maxima on the nanoparticle composition is shown in Fig. 3e . As explained above (equation (2), and its derivation in Methods) for Janus particles, assuming an 'interfacial' layer and a 'bulk' component one expects the peak position to be inversely proportional to the composition. The fit to the data obtained using equation (2) with the interfacial layer thickness t as a parameter provides excellent agreement. In particular, if one treats the data point for Au-DPT 0.19 DDT 0.81 as an outlier, the curve experimental NMR signals can be fitted to a reciprocal functional of y =7.0+6.4/ x ( R 2 =0.976), where y is the NMR chemical shift in p.p.m. and x is the DPT composition. This fit leads to a width of the interfacial ligand layer t of 0.4+/−0.1 nm. To obtain this fit two choices have to be made. The first is the value of the chemical shift I for 'interfacial' signal. This can be either taken by using the intercept to the y axis in Fig. 3d , or by taking the flat region in Fig. 3f , or the first point in Fig. 3e . All these choices have pros and cons, yet they all lead to truly similar fits with equivalent regression values. We chose here the second approach as it provides somewhat a middle value. The value of B was taken from the homoligand particles of the same size. The second choice is whether or not to include the first point (DPT=0.115) in the fit. We decided not to include it as in this case fits became much better. By not including it one gets a t -value of 0.4 nm, the thickness of the DPT calotte for the first point is h =0.3 nm so < t . This provides a (somewhat circular) confirmation of the validity of our choice as for this value of calotte thickness the initial assumption of constant t thickness could have not been met. Following the work of Chen and co-workers, we used NOESY to confirm the Janus nature of these particles. As shown in Fig. 3h (and Supplementary Fig. S9 ), no cross-peaks can be observed in NOESY indicating negligible number of ligands is close to the other kind of ligand. Overall, we can conclude that 1D and 2D NMR clearly show that these particles are of an overall Janus morphology. Striped nanoparticles We synthesized identical nanoparticles to the ones described above with the only difference of being larger (4–5 nm in core diameter). Simulations, and experimental evidences [12] , [13] , [14] , [41] (as well as recent theory on cylindrical surfaces) [42] , [43] , indicate that nanoparticles of this type should have a patchy nature with stripe-like domains for compositions around the 1:1. This happens because the enthalpy of phase separation (that would minimize domain boundaries) is balanced by an interfacial entropy that arise when longer ligands are at an interface with shorter ones (that would tend to maximize interfaces). This entropic contribution is nothing more that extra freedom for the extra length the longer ligands have; it vanishes as particles get smaller and the cone angle that confines a single ligand becomes so large that the whole chain has enough conformational entropy (leading to Janus particles). We have imaged with STM Au-DPT 0.58 DDT 0.42 particles clear stripe-like domains were observed ( Fig. 3l ) [14] . Unlike the results of random particles and Janus particles, the NMR peaks of Au-DPT 0.21 DDT 0.79 and Au-DPT 0.58 DDT 0.42 appear at almost the same position, but that of Au-DPT 0.78 DDT 0.22 clearly shifts to the upfield region. When the DPT content is between 20 and 60%, the centre of the broad aryl peak remains almost the same (green trace, Fig. 3f ), indicating very similar chemical surroundings of DPT molecules. In other words, each DPT molecule has on average the same number of DPT molecules around, although the overall number of DPT ligand per particle increases. When DPT fraction is >60%, a decrease of chemical shift that is caused by the ring current of adjacent DPT molecules is observed (blue trace, Fig. 3f ). This implies the average number of DPT molecules in one DPT molecule's surrounding increases along with the increase of DPT fraction. The significant NOESY cross-peaks observed ( Fig. 3i and Supplementary Fig. S12 ) suggest large amount of interfacial ligands, although the overall sigmoidal shape of 1D NMR indicated phase separation. The combination of these two sets of data can be explained (solely, to the best of our knowledge) by the formation of stripe-like domains. It should be noted that the flat region observed from 20 to 60% DPT implies stripes whose thickness is < 2t . If we assume that t is the same as the one found for the Janus particles of identical composition, that the NMR data imply a stripe width of 0.8±0.2 nm in excellent agreement with the 0.65 nm measured via STM (note that due to the nature of STM experiments, we have always defined stripe thickness as the centre to centre distance between two stripes of equal composition). In addition, we should point out that while STM images show stripe-like domains for Au-DPT 0.58 DDT 0.42 no structure was observed for the Au-DPT 0.78 DDT 0.22 . It is possible that particles from 75 to 100% DPT have a random (or patchy) mixture in their ligand shell. Indeed, one could argue that the trend shown if Fig. 3f in not truly sigmoidal and actually has a linear part that is due to lack of phase separation at those composition. Given the error bars that we have, there is no statistical significance to this observation. In summary, even for this class of particles, we find excellent agreement between the predicted, imaged and NMR determined structures. Data interpretation In a broader sense, when critically analysing the data in Fig. 3f it is possible to see a linear trend were a couple of the points in the 'flat plateau' removed. We notice that each point represents three particles and that for each particle the composition was determined independently via cyanide etching. Yet to be even more certain of our statements, we decided to synthesize different yet similar particles to the ones discussed here. We indeed synthesized particles coated with 1-DDT and TPT. We analysed the particles in the same way as discussed above and we show the results in Fig. 4 . Even though these particles were only synthesized ones, the trend that they show is exactly the one we find for the DPT: DDT particles. The only notable difference is that the flat part is at higher concentrations of the aromatic thiol. Overall, this curve better resembles a polynomial sigmoid. This (with the caveat of the extent of interpretation possible on these curves discussed above) is what one would expect as this longer aromatic should be less miscible with DDT. To further support this interpretation of the curves, we notice that the sharp peaks (discussed below) also linked to phase separation are present in a larger compositional range for these particles. At this point, one might be tempted to use this analysis to at least qualitatively determine the fraction of particles that are stripes/patchy/Janus/mixed. We do not believe that this is possible simply with one technique, but if this technique was to be completed, for example, by mass spectroscopy data and a solid statistical analysis this could be feasible in future. 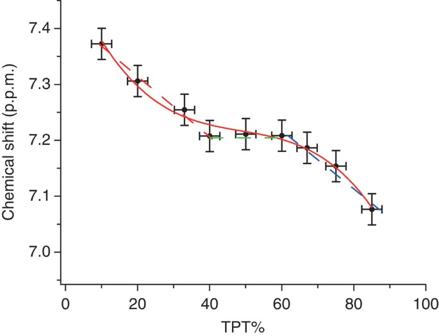Figure 4: Chemical shift of1H NMR as a function of alkanethiol percentage for TPT:DDT striped nanoparticles. Solid red line is the fit to the data. Errors were calculated as average of the s.d. found in general for the composition of all the nanoparticles after cyanide decomposition and for the chemical shift determined for other cases. Figure 4: Chemical shift of 1 H NMR as a function of alkanethiol percentage for TPT:DDT striped nanoparticles. Solid red line is the fit to the data. Errors were calculated as average of the s.d. found in general for the composition of all the nanoparticles after cyanide decomposition and for the chemical shift determined for other cases. Full size image As mentioned earlier, a smaller and sharper NMR peak has been observed at ~7.35 p.p.m. on top of the broad aryl peak of striped particles when the DPT composition was <60%. One may think the sharp peak is from free ligands used for nanoparticle synthesis but not thoroughly removed. We believe that this is not the case for the following two reasons. (a) The peak sustained no matter what methods were used to clean the particles (that is, repeated centrifugation/ultrasonication, filtration and dialysis), and the peak intensity remained the same after additional rounds of cleaning. The absence of any sharp peaks for striped nanoparticles with DPT >60% as well as nanoparticles with Janus and random morphology implies our cleaning methods are effective enough to get rid of excess free ligands. (b) When compared to free DPT, the sharp peaks are still slightly broadened, and no fine structure can be seen. 1 H NMR spectrum of free DPT molecule is composed of a group of peaks with full-width at half-maximum of each being <3 Hz, whereas the full-width at half-maximum of the sharp peak of our nanoparticles is about 16–20 Hz varying on samples and compositions. To further confirm the sharp peak is not due to free ligand, some free ligands were intentionally added to cleaned nanoparticles, and the NMR spectrum of the mixture is significantly different from that of pure nanoparticles ( Fig. 5 ). A new set of small peaks that correspond to free DPT were observed, and the shape and position of the specific sharp peak from nanoparticles remained intact. Moreover, diffusion-ordered spectroscopy NMR was performed on pure nanoparticles, and nanoparticles were mixed with a small amount of free DPT molecules as a control. Diffusion-ordered spectroscopy measures the diffusion coefficient that is related to the hydrodynamic radius of nanoparticles in this study [44] . For our polydispersed nanoparticles, the average diffusion coefficients were calculated using peak intensity at 7.38 (nanoparticles' sharp peak) and 7.58 p.p.m. (DPT's peak furthest from nanoparticles' sharp peak). As calculated by the Stejskal–Tanner equation [45] , ligands giving the sharp peak and the broad peak have the same diffusion rate ( D 7.38p.p.m. =1.778×10 −10 and D 7.58p.p.m. =1.827×10 −10 m 2 s −1 ), whereas the average diffusion coefficient becomes larger when free DPT is mixed ( D ′ 7.38p.p.m. =2.624×10 −10 and D ′ 7.58p.p.m. =3.723×10 −10 m 2 s −1 ). A possibility for the sharp peak is that it arises from certain aryl hydrogen of DPT, most possibly the terminal one which is the furthest from the particle surface, because peaks are less broadened when the nuclei are further away from the diamagnetic layer at the ligand–nanoparticle interface [37] . But this hypothesis cannot explain the fact that the sharp peak is observed on nanoparticles only with stripe morphology but not with Janus or random morphology. Overall, we can conclude the sharp peak that has been reproducibly observed is a real signal of DPT ligands chemically bonded to the nanoparticle surface. 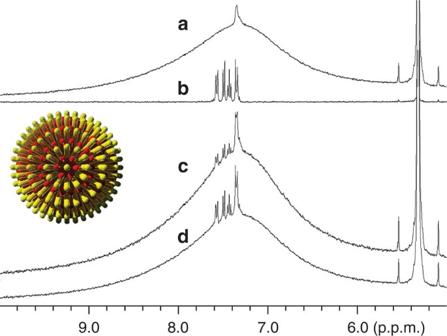Figure 5:1H NMR of striped nanoparticles with addition of a small amount of free DPT. (a) Purified nanoparticles; (b) free DPT ligand; (c) nanoparticles mixed with DPT; (d) nanoparticles mixed with more DPT. Inset shows the defect site (the pole) of striped nanoparticles from a top view. Figure 5: 1 H NMR of striped nanoparticles with addition of a small amount of free DPT. ( a ) Purified nanoparticles; ( b ) free DPT ligand; ( c ) nanoparticles mixed with DPT; ( d ) nanoparticles mixed with more DPT. Inset shows the defect site (the pole) of striped nanoparticles from a top view. Full size image Bimodal peak separation has been observed by Kohlmann et al . [35] on different gold nanoparticles including tiopronin-, butanethiol- and hexanethiol-coated particles in both 1 H and 13 C NMR spectra. Their observation implied NMR peaks of the same ligands at different binding sites might appear differently. Therefore, we predict the small peak is due to ligands at certain binding sites. As the sharp peak is only observed on striped nanoparticles but not on Janus and random nanoparticles, it is reasonable to correlate the sharp peak to the stripe morphology. As the NMR integral of the sharp peak is so small, the DPT ligand must be on a very specific singular site. The existence of two chemically addressable polar defect regions in diametrically opposed positions has been previously predicted and experimentally confirmed [46] , [47] , [48] . At this polar position, place-exchange reactions are significantly favored (in one case we have measured a decrease in the standard free energy of reaction of a factor of ~3–10) [46] , [47] , [48] , hence ligands in those regions must be packed in a more loose way, that is, with more free space. Summarizing at the two polar positions, ligands are less ordered and less tightly packed, hence it can be inferred that the sharp peak is possibly caused by the ligand on such pole positions. These are our main reasons. (a) It is known that NMR peaks become broader if ligands are more ordered and well-packed on nanoparticles [34] , [37] , and vice versa , ligands those are more disordered exhibit sharper NMR peaks. The sharp feature of the peaks suggests greater mobility of these molecules compared with that of other ligands in the rest of mixed SAMs. (b) The chemical shift of sharp peaks remained almost the same and is independent of composition ( Supplementary Fig. S13 ). This indicates the ligands that caused the sharp peaks are located in similar environment and are not affected by the ring currents from other DPT molecules when composition changes. (c) The sharp peaks are always in the downfield region compared with the centre of broad peaks of any ligand composition. As it is known that NMR peak shifts to upfield region if ligands are ordered and tightly packed [33] , [37] , we can conclude the sharp peaks arise from ligands that are less ordered or less tightly packed. Given the above reasons, we believe the sharp peak is a unique feature caused by ligands at the pole positions when the particles are encircled by stripe-like domains. As we already found that the ligands on the pole positions are two orders of magnitude more reactive than those in the bulk monolayer toward ligand exchange reaction [46] , [47] , [48] , it was possible to selectively replace the original ligands at these two polar singularities with other ligands to further confirm that the sharp peak is caused by the ligand on the pole positions. Based on the NMR calculation of the number of DPT molecules at the poles, aminoanthracene (five times in excess to the pole molecules) was added to the nanoparticle solution in dichloromethane and stirred at room temperature for 2 h. Then, the nanoparticles were purified by Sephadex column and analysed by NMR. 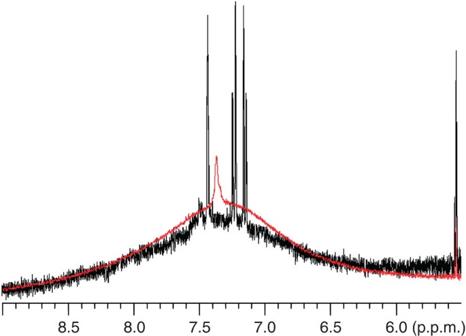Figure 6:1H NMR of nanoparticles. Au-DPT0.27DDT0.73before (red) and after ligand exchange with aminoanthracene (black). Figure 6 shows the 1 H NMR spectra of nanoparticles before and after ligand exchange with aminoanthracene. The original small peak disappeared and a new set of sharp peaks, which is different from those of free aminoanthracene molecules ( Supplementary Fig. S15 ), was observed. The absence of these peaks for homoligand nanoparticles Au-DDT that underwent the same procedure was used as a control and additionally showed that the new peaks were not a result of Sephadex column. This result indicates the original sharp peak on cleaned nanoparticles is from ligands at more reactive binding sites, which we have previously shown to be the polar positions. Figure 6: 1 H NMR of nanoparticles. Au-DPT 0.27 DDT 0.73 before (red) and after ligand exchange with aminoanthracene (black). Full size image Given the finding that the small sharp peak is from ligands on the pole positions, we can use the NMR integrals to estimate the number of pole molecules per particle. Nanoparticles were prepared as a high concentrated solution in 1,1,2,2,-tetrachloroethane- d 2 . The ratio of small peak to the solvent residue peak was calculated by careful deconvolution via Gaussian–Lorentzian fitting (see Supplementary Fig. S16 as an example). Then, the particles were heated at 75 °C for a week in a perfectly sealed NMR tube to completely release all ligands from particle surface, so the peak for overall DPT is no longer broad and can be accurately integrated (see Supplementary Fig. S17 as a representative 1 H NMR spectrum of samples after thermal decomposition). Under the assumption of no loss of solvent molecules as it has a high boiling point at 145 °C, we are able to use the integrals of solvent residue peak as a reference to study the relative ratio of the pole ligands, overall DPT ligands and DDT ligands. Nanoparticles with a few different compositions have been measured and the number of pole molecules per particle is listed in Table 2 . Even though the DPT percentage changes from 26 to 40%, the number of DPT ligand at the pole positions remains the same (that is, within the error in the measurement), further confirming our interpretation for these peaks. Table 2 Average number of DPT ligand at pole positions per particle. Full size table In conclusion, we have shown that a combination of 1D and 2D NRM can be used to determine the ligand shell morphology of gold nanoparticles coated with binary mixtures of aromatic and aliphatic ligand molecules. We predict and experimentally show that for randomly mixed ligand shells there is a linear dependence of the aromatic hydrogens peak position over the particles composition with the presence of clear cross-peaks in the NOESY spectra. For Janus particles, the linear dependence becomes a 1/ x dependence and the cross-peaks in the NOESY spectra disappear. In the case of patchy particles, we observe a sigmoidal dependence with cross-peaks reappearing in the NOESY spectra. In the stripe range of composition, we observe an overall constant peak position that we explain with the stripe width being less than or equal to two interfacial layers. Given that we can obtain the thickness of this layer from the analysis of Janus particles of identical composition but smaller size, we can estimate the stripe thickness to be 0.8±0.2 nm, which is in excellent agreement with the one measured via STM. Furthermore, we have shown that the 1D NMR spectra of striped (and only striped) nanoparticles shows the presence of somewhat sharp peaks that we can assign to molecules being at the polar defect regions characteristic of striped nanoparticles. Overall, NMR is a simple and fast method that can be conducted in most laboratories in the world. Here, we have shown that it can be used to study the morphology of mixed ligands on nanoparticles. We believe that this approach could be used to uniquely identify ligand shell morphology of mixed ligands in nanoparticles and other nanomaterials. At present, the main limitation of this method is that of needing one ligand to contain an aryl group, with the aromatic peak well separated from the peaks of the other molecules. We realize that this is a serious limitation, yet this remains a powerful method to analyse the ligand shell structure for this family of particles. Another limitation stands in the fact that a whole series of particles (possibly with each composition synthesized multiple times) needs to be investigated before reaching a conclusion on the ligand shell morphology. Furthermore, when particles become too large we expect the signal to be too weak to be analysed. We should point out that for smaller nanoparitlces other NMR-based approaches for the analysis of the ligand shell have been developed [49] , [50] . The future of this field will be in the determination of the fraction of sample that is patchy versus striped versus Janus or mixed, as well as in the characterization of the exact quality of the patchiness of samples. This, we believe, will not come from a single technique rather from a combination of techniques. General DPT was purchased from Oakwood Products, Inc. All other chemicals were purchased from Sigma-Aldrich and used as received. Nanoparticles' average core size was determined using TEM images captured by JEOL 200CX at 200 kV or Philips CM20 at 120 kV. The STM experiments were performed at room temperature using a Veeco Multimode Scanning Probe Microscopy with E scanner in an acoustic chamber sitting on a vibration-damping table in air. Mechanically cut Platinum-iridium STM tips were used. Set point currents were in the range of 40–80 pA with a voltage bias of 800–1,300 mV. NMR solutions of nanoparticles were prepared in CD 2 Cl 2 or C 2 D 2 Cl 4 at about 5 mg ml −1 . Spectra were obtained using a Bruker 400 MHz spectrometer and referenced to the solvent peak of dichloromethane- d 2 at 5.32 ppm and for tetrachloroethane- d 2 at 6.00 ppm. Standard Bruker NOESY setting was used for the experiment. D1 delay time was set to 2 s, and D8 mixing time was set to 400 ms. Number of scans was 16. Derivation for equation 2 To calculate the composition dependence of the peak F for a generic hydrogen on a Janus particle, we made the following assumptions. First, we assumed that all the ligand molecules pack in the same way. This implies that ligand A will occupy a calotte on the sphere of area A =2 πrh , with r being the radius of the core of the particles and h being the height of the calotte (that is the fraction of the radius perpendicular to the plane of the calotte that starts at the surface of the sphere and end at the intercept with the callotte's plane). Given the fist assumption it is trivial to derive the following relation: x A = h /2 r . We then assume that the signal F is a linear combination of the signal coming from an interfacial layer whose thickness t does not depend on composition and the signal coming from a bulk layer that is far enough from the interface so that its F is the same of that of homoligand nanoparticles. The F of the former we call I , the one of the latter we call B . It is immediate that the 'bulk' layer will occupy a calotte of height h′ with the following relation holding: h = h′ + t . The area of the interfacial ring will be: A I =2 πrt . Using the second assumption we get that . Synthesis of 4–5 nm Au-DPT x DDT 1− x Stock solutions of triphenylphosphinegold(I) chloride (0.060 mmol ml −1 ), DPT (0.020 mmol ml −1 ), DDT (0.020 mmol ml −1 ) and boran t–butylamine complex (1.2 mmol ml −1 ) were prepared in dichloromethane right before use. In a 50-ml round bottom flask, 4.0 ml solution of triphenylphosphinegold(I) chloride was mixed with 6.0 ml the solution of thiol mixture. The mixture was stirred at room temperature for 30 min. Then, 9 ml dichloromethane and 2.0 ml borane t–butylamine complex solution was added sequentially. The reaction mixture was stirred at room temperature for 5 h. A volume of 25 ml methanol was added to quench the reaction and precipitate nanoparticles. Nanoparticles were stored at 4 °C overnight, purified by repeated centrifugation and ultrasonication, and stored as solution in dichloromethane at −10 °C. Synthesis of ~2 nm Au-DPT x DDT 1− x The synthesis of ~2 nm Au-DPT x DDT 1− x followed the same protocol of the synthesis of 4–5 nm Au-DPT x DDT 1− x , but the reactions were quenched at 20 min after the addition of borane t–butylamine complex. Synthesis of 4–5 nm Au-DPT x DMOT 1− x The branched octanethiol ligand (DMOT), 3,7-dimethyl-1-octanethiol, was synthesized as previously reported (ref. 16 ). The synthesis of 4–5 nm Au-DPT x DMOT 1− x followed the same protocol of the synthesis of 4–5 nm Au-DPT x DDT 1− x . Etching Nanoparticles in dichloromethane (5 mg ml −1 ) were mixed with an aqueous solution of sodium cyanide (1.0 M) in a 1:1 volume ratio. The mixture was stirred at room temperature, exposed to air, until the organic layer turned colourless or light yellow. The organic layer was separated and washed with an equal volume of water (three times). How to cite this article: Liu, X. et al . Determination of monolayer-protected gold nanoparticle ligand-shell morphology using NMR. Nat. Commun. 3:1182 doi: 10.1038/ncomms2155 (2012).